Metal single-site catalyst design for electrocatalytic production of hydrogen peroxide at industrial-relevant currents Direct hydrogen peroxide (H 2 O 2 ) electrosynthesis via the two-electron oxygen reduction reaction is a sustainable alternative to the traditional energy-intensive anthraquinone technology. However, high-performance and scalable electrocatalysts with industrial-relevant production rates remain to be challenging, partially due to insufficient atomic level understanding in catalyst design. Here we utilize theoretical approaches to identify transition-metal single-site catalysts for two-electron oxygen reduction using the *OOH binding energy as a descriptor. The theoretical predictions are then used as guidance to synthesize the desired cobalt single-site catalyst with a O-modified Co-(pyrrolic N) 4 configuration that can achieve industrial-relevant current densities up to 300 mA cm − 2 with 96–100% Faradaic efficiencies for H 2 O 2 production at a record rate of 11,527 mmol h − 1 g cat − 1 . Here, we show the feasibility and versatility of metal single-site catalyst design using various commercial carbon and cobalt phthalocyanine as starting materials and the high applicability for H 2 O 2 electrosynthesis in acidic, neutral and alkaline electrolytes. Hydrogen peroxide (H 2 O 2 ) has been widely used in industrial processes including in fiber and paper production, water treatment and environmental remediation in acidic and neutral mediums [1] , [2] , [3] , [4] . Currently, commercial H 2 O 2 manufacture primarily relies on the large-scale anthraquinone oxidation process; however, this technology requires enormous capital input for infrastructure, and is energy-intensive accompanied by substantial quantities of hazardous waste discharge during operation. In order to minimize the transportation cost from manufacturing point to end-users, H 2 O 2 is concentrated up to 70 wt%, which poses safety issues due to potential explosion risk and brings about extra carbon footprint. Additionally, the addition of stabilizers to prevent H 2 O 2 degradation often negatively affects the chemical activity of H 2 O 2 , while the chemical residues also create concerns in water treatment applications. Thus, it is highly desired to realize sustainable production of H 2 O 2 using electric energy that would enable portable and safe on-demand H 2 O 2 supply for decentralized or remote locations. Recent advances demonstrate that the electrocatalytic two-electron oxygen reduction reaction (ORR) with H 2 O and O 2 as reactants provides a promising route for direct H 2 O 2 production [1] , [5] , [6] , [7] , [8] . Carbonaceous catalysts show high two-electron ORR selectivity but a low intrinsic activity compared to metal-based catalysts due to weak *OOH binding [9] , [10] . Platinum-group metals are recognized as the most active ORR catalysts [11] , [12] , [13] , but for exclusive four-electron pathway to H 2 O due to the strong *OOH binding on adjacent metal atoms to cause O–O breakage. Theoretically, the activity and selectivity of the two-electron ORR follow the Sabatier volcano-type dependence on the *OOH binding, where the optimal performance can be achieved with a suitable *OOH binding energy that situates at the volcano peak [11] , [14] , [15] . Stephens and Rossmeisl, et al. proposed the spatial site isolation strategy of reactive metal atoms using inert Au or Hg elements, and discovered the PtHg 4 alloy with outstanding electrocatalytic property for H 2 O 2 production by computational screening using the density functional theory (DFT) method [14] . Chorkendorff and Stephens, et al. identified Ag−Hg and Pd−Hg catalysts highly active and selective for H 2 O 2 production by searching the optimal *OOH binding closest to the volcano peak [15] . Therefore, the theoretically calculated two-electron ORR volcano plot with the *OOH binding as the descriptor can be regarded as one effective tool to discover new catalysts for H 2 O 2 electrosynthesis by computational screening. Metal single-site catalysts (SSCs) have the isolated and active sites with the adjustable electronic property by regulating the metal centers and the coordination configurations, which provides the opportunities for the *OOH binding tuning [5] , [6] , [16] . Recent studies indicate that the transition-metal SSCs, such as Co, Fe and Ni, show the electrocatalytic activities for H 2 O 2 production [3] , [17] , [18] , [19] , [20] . For example, iron single atoms coordinated with C and O atoms exhibited high H 2 O 2 selectivity, in contrast to the well-known FeN 4 for H 2 O formation [3] , [21] . The Co SSCs have attracted extensive attentions due to the more suitable *OOH binding for H 2 O 2 production, however, the widely known CoN 4 are less selective for H 2 O 2 due to the strong *OOH binding [18] . It was reported that introducing the oxygen-containing groups around the CoN 4 sites could weaken *OOH binding and enhance the H 2 O 2 selectivity [17] , [18] , [19] . However, the electronic effects induced by configurational variation of the active metal moiety and the atomic level modification mechanisms still remain insufficiently understood for the two-electron ORR. Moreover, it is often difficult to achieve scalable synthesis of well-defined SSCs with atomic level control due to the inhomogeneity and the random dispersion of metal sites. The practical electrocatalytic H 2 O 2 synthesis still faces great challenges of achieving both commercially relevant currents and H 2 O 2 Faradaic efficiency (FE), which is often characterized by low H 2 O 2 production rate and product concentration. Thus, it is critical to develop implementable design for developing high-performance and low-cost two-electron ORR catalysts for high-efficiency H 2 O 2 electrosynthesis. Here, we report oxygen groups modified transition-metal phthalocyanine (TMPc) catalysts with TM-(pyrrolic N) 4 configuration for high-performance H 2 O 2 synthesis in acidic, neutral and alkaline electrolytes. The electronic properties of TMPc are adjusted by changing the metal centers and the adjacent coordination atoms from oxidized carbon nanotube (OCNT) support, thus enhancing the H 2 O 2 selectivity. DFT calculations are conducted to screen for highly selective and active two-electron ORR electrocatalysts among TMPc catalysts by establishing the activity-volcano plot with the *OOH binding energy as the descriptor. The optimal *OOH binding at the volcano peak is achieved for cobalt phthalocyanine molecule anchored on oxygen-modified carbon plane (CoPc-OCNT), which can be ascribed to the electronic state modification below the Fermi level. The prepared CoPc-OCNT catalyst shows the high activity and exclusive selectivity for H 2 O 2 electrosynthesis in alkaline electrolyte, where the industrial-relevant current density up to 300 mA cm − 2 is achieved at a remarkable production rate while maintaining high FE. The CoPc-OCNT catalyst also obtains good H 2 O 2 electrosynthesis performance using a neutral or acidic electrolyte, which is applicable for wastewater treatment. It also demonstrates the versatility of designing oxygen groups modified Co SSCs for H 2 O 2 electrosynthesis by employing a variety of commercial carbon materials, showing the promising potential in scalable catalyst preparation. Theoretical calculations DFT calculations are conducted to screen for highly active and selective two-electron ORR electrocatalyst among TMPc including MnPc, FePc, CoPc, NiPc, CuPc and ZnPc (Fig. 1a and Supplementary Figs. 1 , 2 ). 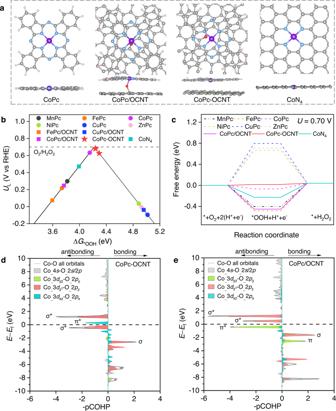Fig. 1: Theoretical calculations for two-electron ORR. aAtomic structures of CoPc, CoPc/OCNT, CoPc-OCNT and CoN4models.bCalculated activity-volcano curve for two-electron ORR.cFree-energy diagrams for two-electron ORR pathway at 0.7 V vs RHE, where * and *OOH denote an unoccupied active site and adsorbed *OOH, respectively.d–eProjected crystal orbital Hamilton populations (pCOHP) between Co and p-orbital of O of *OOH on CoPc/OCNT and CoPc-OCNT. Figure 1b shows the volcano plot describing the two-electron ORR activity as a function of the Gibbs free energy for *OOH adsorption (Δ G *OOH ). MnPc and FePc, situated on the left side of volcano plot, show strong *OOH binding to favorably dissociate the O–O bond adsorbed on active metal sites, resulting in selective H 2 O formation over H 2 O 2 [14] , [15] . NiPc, CuPc and ZnPc, located at the right side, present weak *OOH binding and thus high selectivity to H 2 O 2 formation; however, the ORR activities are proposed to be inferior due to the rate-limiting protonation of O 2 toward *OOH. In contrast, CoPc shows a Δ G *OOH value of 4.15 eV that is closest to the activity-volcano peak (~4.22 eV) [14] , demonstrating the highest activity and selectivity toward the two-electron ORR among all TMPc assessed here. Free energy diagrams for the two-electron ORR in Fig. 1c display the largely uphill barrier, up to 0.66–0.80 eV, to form the *OOH intermediate on NiPc, CuPc and ZnPc at 0.7 V, confirming the poor ORR activities. In contrast, the energy barrier of 0.40–0.48 eV for *OOH dissociation on both MnPc and FePc, originated from the excessively downhill step to form the *OOH, would drastically reduce the selectivity to H 2 O 2 . In line with the activity-volcano relationship, CoPc shows the lowest energy barrier of 0.07 eV for the entire reaction process of oxygen reduction to H 2 O 2 formation, although there is still a small energy gap to the ideal reaction process where the free energy change is flat with zero energy barrier [11] , [15] . It is worth noting that the Δ G *OOH values of MnPc, FePc, CoPc, NiPc and CuPc show the correlation with the d-band center (Supplementary Figs. 3 , 4 ), where the lower d-band center of metal atoms contributes to more positive Δ G *OOH and thus weaker binding ability [22] , [23] . Furthermore, the adjustment of adjacent atomic environment of the metal sites can also effectively optimize the *OOH binding by modifying the electronic structures [17] , [18] , [19] . Compared to CoPc, the too strong *OOH binding away from the top of the volcano plot on the typical CoN 4 structure suggests the possibility of tuning ORR selectivity by coordinating the Co center. The O-modified graphitic carbon is employed to anchor the CoPc molecule for modifying the local configuration of the Co center. It’s worth noting that O modified graphitic carbon have poor ORR activity due to weak *OOH binding, while the Co site of CoPc has good *OOH binding and is highly ORR active that can be ascribed to the high electrophilicity to *OOH (Supplementary Figs. 5 – 7 ). Interestingly, it is found that different types of O atoms on the carbon plane (Supplementary Fig. 8 ) result in two opposite effects that strengthen or weaken the *OOH binding on CoPc. The O dopant at the defective carbon site helps the Co site (denoted as CoPc-OCNT) achieve a slightly increased Δ G *OOH that is closest to the activity-volcano peak (Fig. 1b ). The corresponding free energy diagram exhibits a negligible uphill energy barrier (Fig. 1c ), suggesting excellent two-electron ORR activity of CoPc-OCNT. However, axial O coordination at the carbon basal plane to the Co center (denoted as CoPc/OCNT) causes a stronger *OOH binding with a reduced Δ G *OOH of 3.77 eV and increases the energy barrier (0.45 eV) for H 2 O 2 formation, adversely reducing the two-electron selectivity. The effect of axial O coordination is also confirmed on FePc or CuPc, which causes stronger *OOH binding and thus lower H 2 O 2 selectivity on Fe site while moderately improved ORR activity on Cu site (Supplementary Fig. 9 ). We further examine the H 2 O 2 selectivity of catalysts by inspecting the entire ORR process containing three primitive steps of *+O 2 →*OOH→*H 2 O 2 →*+H 2 O 2 as well as the O‒O bond dissociation of the adsorbed *OOH or *H 2 O 2 (Supplementary Fig. 10 ). The CoPc-OCNT catalyst shows a small energy barrier during the entire two-electron ORR process, indicating a low overpotential for producing H 2 O 2 . It is important to note that the thermodynamically favorable O‒O bond breakage via the dissociation of *H 2 O 2 or *OOH over H 2 O 2 formation does not imply a low H 2 O 2 selectivity as the kinetic energy barrier under real electrocatalytic conditions is likely high enough to prevent the O‒O from breaking [24] , [25] (see more analysis in Supporting Information). To bridge the gap between the theoretical models and real catalytic configurations, several types of possible OCNT structures with O dopant locating at different defective sites are considered as the supports of CoPc (shown in Supplementary Fig. 11 ). They show similar Δ G *OOH values, suggesting that the C‒O‒O group at the defective site can effectively modify the Co sites of CoPc to achieve an optimal *OOH binding energy. Furthermore, we find that cobalt tetrabenzoporphyrin (CoTBP) with four pyrrolic N coordination supported by OCNT also show the optimal *OOH binding energy that is close to the peak of the volcano (Supplementary Fig. 12 ). Thus, we infer that Co sites of these Co SSC coordinated with pyrrolic N are intrinsically active to selectively catalyze two-electron ORR. Fig. 1: Theoretical calculations for two-electron ORR. a Atomic structures of CoPc, CoPc/OCNT, CoPc-OCNT and CoN 4 models. b Calculated activity-volcano curve for two-electron ORR. c Free-energy diagrams for two-electron ORR pathway at 0.7 V vs RHE, where * and *OOH denote an unoccupied active site and adsorbed *OOH, respectively. d–e Projected crystal orbital Hamilton populations (pCOHP) between Co and p-orbital of O of *OOH on CoPc/OCNT and CoPc-OCNT. Full size image To uncover the origin for ORR selectivity tuning on Co SSC, the electronic properties of the Co atom in CoPc/OCNT and CoPc-OCNT are analyzed by studying the density of states and Bader charge. Projected density of states (PDOS) of CoPc/OCNT and CoPc-OCNT in Supplementary Fig. 13 reveal that the different degree of orbital hybridization before and after *OOH adsorption determine the properties of *OOH adsorption. We calculate the projected crystal orbital Hamilton populations (pCOHP) between the Co atom and the O atom of *OOH to explain the bond strength (Fig. 1d ). The pCOHP of CoPc/OCNT shows that all antibonding σ* orbitals are located at unoccupied states above the Fermi level, which contributes to reinforced *OOH adsorption. In contrast, pCOHP of CoPc-OCNT reveals that antibonding electrons of the σ* orbital with highly occupied states below the Fermi level reduce the strength of the Co‒O bond, which well accounts for weaker *OOH adsorption. Moreover, the absence of the back-donation effect due to antibonding π* with unoccupied state above the Fermi level is also responsible for the weak Co‒O bond in CoPc-OCNT. Bader charge analysis indicates charge loss at the Co site and charge accumulation at the O atom after *OOH is adsorbed (Supplementary Figs. 14 , 15 and Supplementary Table 1 )), suggesting charge transfer from the Co center to O atoms. More charge lose on Co atom in CoPc-OCNT (−0.898 | e |) compared with CoPc (−0.898 | e |) and CoPc/OCNT (−0.612 | e |) suggests the intensified electron transfer from Co to surrounding ligands (Supplementary Figs. 16 , 17 ), which is responsible for the weaker *OOH binding. Metal single-site catalyst synthesis and characterization Guided by the theoretical predictions, TMPc-OCNT (TM=Fe, Co or Cu) catalysts are synthesized by combining TMPc with the OCNT support through a sufficient mixing process (see Methods). This mild synthetic method at room temperature is adopted to avoid generating the strong bonding between the TM site in TMPc and the O atom in OCNT and to prevent the decomposition of TMPc molecules in typical high-temperature processing. The OCNT material is prepared by oxidatively treating the original CNT (ori-CNT) to create oxygen-containing functional groups. As illustrated in Supplementary Fig. 18 , no visible morphology changes are observed on OCNT after oxidation. X-ray photoelectron spectroscopy (XPS) measurements show that OCNT has a significantly increased O content (9.1%) compared to ori-CNT (2.5%), and these introduced oxygen functional groups exist mainly in the form of C–O–C (O at defective site) as well as minor portion of C=O (O on carbon plane) [18] , [26] , as also revealed by Fourier transform infrared (FT-IR) spectra (Supplementary Fig. 19 ). Raman spectra reveal an obvious increasement of carbon defects in OCNT due to more O dopant. The analysis of N 2 adsorption-desorption isotherms shows a two-fold increase in the specific surface area of OCNT compared to ori-CNT (Supplementary Fig. 20 ), which is favorable to provide more opportunities to anchor TMPc molecules. The atomic contents of Fe, Co and Cu are determined by XPS to be 0.57, 0.30 and 0.79 at% on the surface of FePc-OCNT, CoPc-OCNT and CuPc-OCNT, respectively, (Supplementary Fig. 21 ). The X-ray diffraction (XRD) patterns show that all TMPc-OCNT catalysts contain the characteristic diffraction peaks that are well-matched with reference TMPc molecules (Supplementary Fig. 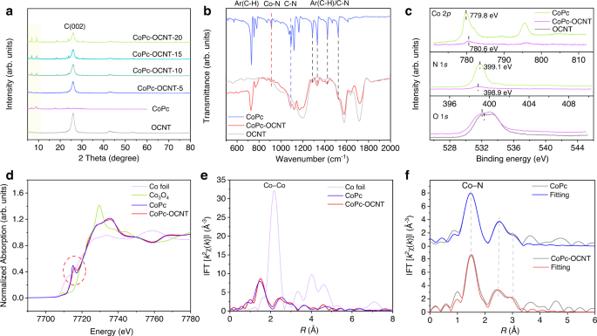Fig. 2: Characterizations of Co sites in the CoPc-OCNT catalyst. aXRD patterns of CoPc-OCNT with different Co loadings.bFT-IR spectra of OCNT, CoPc-OCNT and CoPc reference.cCo 2p, N 1sand O 1shigh-resolution XPS spectra of CoPc-OCNT and the reference materials (Co foil, Co3O4and CoPc).dXANES ande–fFT-EXAFS curves atRspace of Co K-edge and the corresponding fittings for CoPc-OCNT and the reference materials (Co foil and CoPc). 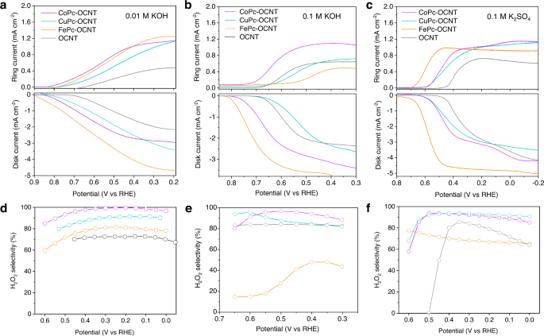Fig. 3: Two-electron ORR activity and selectivity evaluation of the TMPc-OCNT catalysts using RRDE. Linear sweep voltammetry show that ORR and simultaneous H2O2oxidization currents are achieved on disk and ring electrodes, respectively.a-bTests in 0.01 M KOH (pH 11.9)c-d0.1 M KOH (pH 12.7) ande-f0.1 M K2SO4(pH 7.2). 22 ), suggesting that the molecular structures of TMPc are retained after being anchored on OCNT. The XRD patterns for CoPc-OCNT (Fig. 2a ) show that the characteristic peaks located at 7.0° and 9.2° are markedly increased in intensity when the CoPc content is increased from 0.23 to 0.45 at% (Supplementary Tables 2 , 3 ) [27] , indicating that the loading of molecular CoPc can be adjustable by increasing concentration. The FT-IR results of CoPc-OCNT display the characteristic vibrational peaks located at 435–873, 915 and 1090–1524 cm − 1 that are assigned to the C–H/C–C bending, Co–N and C–H/C–N stretching (Fig. 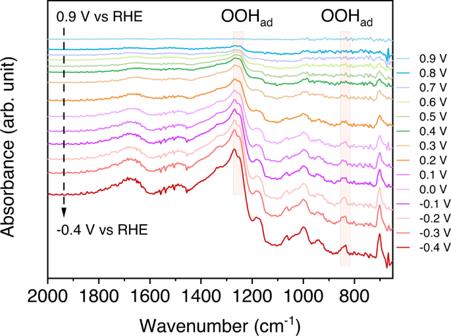Fig. 4: In situ detection of *OOH species. In situ ATR-SEIRAS spectra collected on CoPc-OCNT catalyst in O2-saturated 1.0 M KOH catholyte at different potentials from 0.9 to −0.4 V vs RHE (OOHad: adsorbed *OOH). 2b and Supplementary Table 4 ), respectively, being in good agreement with the CoPc reference and confirming the undamaged molecular CoPc structure anchored on OCNT [27] , [28] . Similar results are also observed on CuPc-OCNT and FePc-OCNT (Supplementary Fig. 23 ), indicating the successful CuPc and FePc loading. Furthermore, we examine the chemical interactions between Co of CoPc and O of the OCNT by high-resolution XPS spectra, which reveals a slight peak shift in the Co peak of CoPc-OCNT to higher binding energy comparing to CoPc, which is companied by a reverse shift of the O peak (Fig. 2c ). Similar shifts of spectral peaks are also observed on FePc-OCNT and CuPc-OCNT but not on Pc-OCNT (Supplementary Fig. 24 ), indicating more positive valence for the metal sites, likely due to charge transfer from the metal centers to surrounding coordinated atoms [29] , [30] , [31] , [32] . Additionally, the O 1 s high-resolution spectrum reveals that the C–O–C group is dominant in CoPc-OCNT compared to C=O. To identify the structural configuration of metal sites in CoPc-OCNT, X-ray absorption near edge spectroscopy (XANES) and extended X-ray absorption fine structure (EXAFS) of the Co K-edge are analyzed. As illustrated in Fig. 2d , the near-edge absorption intensity of the Co K-edge for CoPc-OCNT is between that of Co foil and Co 2 O 3 , suggesting a positively charged Co atom [32] , [33] . The detection of the pre-edge peak at 7715 eV (a signature of the square-planar Co–N 4 structure in CoPc) indicates that the configuration of Co–N 4 remains intact on OCNT [33] , [34] , [35] . Referring to the Fourier transformed EXAFS (FT-EXAFS) for Co foil (Fig. 2e and Supplementary Fig. 25 ), the Co–Co scattering path (2.2 Å) is absent in CoPc-OCNT, indicating that Co exists as isolated single sites. In comparison with CoPc, the EXAFS fitting for CoPc-OCNT shows a main peak at 1.5 Å and the minor peaks at 2.5 and 3.0 Å that can be assigned to the first scattering path of Co–N and the second paths of Co–C–N and Co–N–C, respectively (Fig. 2f ). The quantitative fitting of the EXAFS spectra reveals the first coordination shell of four Co–N bonds at the distance of 1.9 Å and the second shell of Co–N–C and Co–C–N at the distances of 3.3 and 3.0 Å (Supplementary Fig. 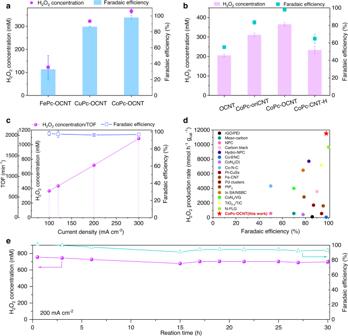Fig. 5: H2O2electrosynthesis performance in a flow-cell electrolyzer based on the gas-diffusion cathode. a, bConcentrations of H2O2directly outputted from electrolyzer and the Faradaic efficiency of FePc-OCNT, CoPc-OCNT, CuPc-OCNT, OCNT, CoPc-oriCNT or CoPc-CNT-H cathodes at 100 mA cm−2(Data points and error bars represent the average and standard deviation of data from triplicate parallel tests).cH2O2concentration, Faradaic efficiency and TOF values of CoPc-OCNT at 100, 120, 200 and 300 mA cm−2.dH2O2production rate of CoPc-OCNT compared with most advanced catalysts newly reported (data sources are provided in Supplementary Table8).eStability evaluation of CoPc-OCNT cathode for continuous electrosynthesis of H2O2at 200 mA cm−2in a chronopotentiometry test. (Cathodic working area of 1 cm−2, the catholyte of 1.0 M KOH (pH 13.7) is one-pass flowed out at a rate of 5 mL h−1to bring out the generated H2O2, while the anolyte of 0.5 M H2SO4was circled at a rate of 33 mL h−1). 26 and Supplementary Table 5 ). Overall, the results above reveal the CoPc-like Co-(pyrrolic N) 4 structure with O atom modification in CoPc-OCNT. Fig. 2: Characterizations of Co sites in the CoPc-OCNT catalyst. a XRD patterns of CoPc-OCNT with different Co loadings. b FT-IR spectra of OCNT, CoPc-OCNT and CoPc reference. c Co 2 p , N 1 s and O 1 s high-resolution XPS spectra of CoPc-OCNT and the reference materials (Co foil, Co 3 O 4 and CoPc). d XANES and e–f FT-EXAFS curves at R space of Co K-edge and the corresponding fittings for CoPc-OCNT and the reference materials (Co foil and CoPc). Full size image Electrocatalytic two-electron ORR performance The two-electron ORR activity and selectivity of TMPc-OCNT catalysts are investigated by rotating ring-disk electrode (RRDE) using a standard three-electrode system in 0.01 M KOH (pH 11.9), 0.1 M KOH (pH 12.7) and 0.1 M K 2 SO 4 (pH 7.2) electrolytes. Catalyst is precisely casted on the disk region for catalyzing ORR to H 2 O 2 , and as-generated H 2 O 2 is detected by the Pt ring electrode. The ORR and H 2 O 2 oxidation currents in Fig. 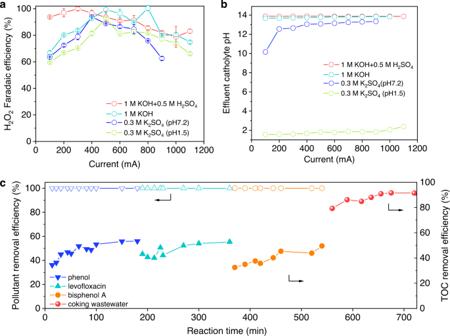Fig. 6: Acidic electrosynthesis H2O2performance and Fenton applications. a, bH2O2electrosynthesis employing 1 M KOH+0.5 M H2SO4, 1 M KOH+1 M KOH, 0.3 M K2SO4+0.3 M K2SO4(pH 7.2 or 1.5) as catholyte and anolyte in the bigger flow-cell electrolyzer (test conditions: cathodic working area of 4 cm−2, catholyte and anolyte flow rates of 82–100 mL h−1).cPollutant removal and TOC removal efficiency by the flow-cell Fenton system. (Test conditions: 500 mA current, effluent H2O2rate of 72 mL h−1synthetic wastewater: 10 mg  L−1phenol, bisphenol A or levofloxacin and 1 mM Fe2+, flow rate of 700 mL h−1real coking wastewater: initial TOC of 44.1 mg L−1, 5 mM Fe2+dosage, flow rate of 140 mL h−1.). 3a exhibit that TMPc-OCNT catalysts show better activity with a more positive onset potential of 0.75–0.81 V vs RHE (defined at −0.1 mA cm − 2 of H 2 O 2 partial current) [36] compared with OCNT (0.71 V vs RHE) in 0.01 M KOH (Supplementary Table 6 ). The negligible overpotentials on TMPc-OCNT for the two-electron ORR compared to the standard equilibrium potential of 0.76 V vs RHE in less alkaline solution suggests fast kinetics. Significantly, CoPc-OCNT exhibits the highest H 2 O 2 selectivity of 95–100% in the potential range of 0–0.45 V vs RHE that is higher than that on CuPc-OCNT (86–91%), FePc-OCNT (75–81%) and OCNT (70–61%) (Fig. 3b ). In 0.1 M KOH electrolyte, CoPc-OCNT also exhibits the highest H 2 O 2 selectivity and activity among all tested catalysts (Fig. 3c, d ). Noting that CuPc-OCNT shows a high H 2 O 2 selectivity but lower activity, while FePc-OCNT has the opposite ORR performance, which is consistent with the theoretical predictions as aforementioned. Similar performance trends of catalysts are also observed in the neutral electrolyte of 0.1 M K 2 SO 4 (Fig. 3e, f ), and TMPc-OCNT catalysts show smaller overpotentials and higher H 2 O 2 partial current densities compared with OCNT. Overall, CoPc-OCNT shows the best H 2 O 2 activity and H 2 O 2 partial current density in both alkaline and neutral conditions, being consistent with the theoretically predicted best performance from the volcano plot based on Δ G *OOH . The experimentally observed potential- or pH-dependent ORR activity and H 2 O 2 selectivity are related with kinetics in electrocatalytic solid−liquid interfaces, which can be further explained by the simulation of kinetics involving water layers using advanced dynamic models [24] , [25] . Fig. 3: Two-electron ORR activity and selectivity evaluation of the TMPc-OCNT catalysts using RRDE. Linear sweep voltammetry show that ORR and simultaneous H 2 O 2 oxidization currents are achieved on disk and ring electrodes, respectively. a-b Tests in 0.01 M KOH (pH 11.9) c-d 0.1 M KOH (pH 12.7) and e-f 0.1 M K 2 SO 4 (pH 7.2). Full size image In situ attenuated total reflectance surface-enhanced infrared absorption spectroscopy (ATR-SEIRAS) testes are performed to detect the key adsorbed OOH* on CoPc-OCNT during the electrolytic H 2 O 2 synthesis (Supplementary Fig. 27 ). Figure 4 shows that a weak absorption band at about 1264 cm − 1 appears when applying a potential of 0.8 V vs RHE, and this band is gradually enhanced by decreasing the potential. These absorption band on CoPc-OCNT can be assigned to O–O stretching vibration of *OOH, which are slightly shifted to higher wavenumber compared with the values in previous studies likely due to different adsorption sites [17] , [37] , [38] . Additionally, the bands at 835 cm − 1 that increase with negatively shifted potential can be reasonably assigned to the M–O stretching mode of *OOH [39] , [40] , [41] . Moreover, the bands assigned to adsorbed hydroperoxide (typically at 1386 cm − 1 ) are not detected [37] , because H 2 O − product rather than H 2 O 2 is produced at pH>11.6. Overall, the detection of the potential-dependent adsorbed hydroperoxy bands supports the *OOH mediated two-electron ORR pathway on the CoPc-OCNT catalyst. Fig. 4: In situ detection of *OOH species. In situ ATR-SEIRAS spectra collected on CoPc-OCNT catalyst in O 2 -saturated 1.0 M KOH catholyte at different potentials from 0.9 to −0.4 V vs RHE (OOH ad : adsorbed *OOH). Full size image To evaluate the ability for electrocatalytically producing H 2 O 2 , the CoPc-OCNT catalyst is deposited on hydrophobic gas-diffusion electrode for enhancing O 2 supply. We employ a two-electrode system assembled in a customized flow-cell reactor, as illustrated in Supplementary Fig. 28 . As shown in Fig. 5a , the CoPc-OCNT can continuously produce 366 mM H 2 O 2 solution with 98% FE at 100 mA cm − 2 , which is significantly greater than CuPc-OCNT (322 mM, 86%) and FePc-OCNT (123 mM, 33%). The H 2 O 2 FE on both CoPc-OCNT and CuPc-OCNT are close to that measured by RRDE, suggesting high H 2 O 2 selectivity and weak activity in decomposing H 2 O 2 . It is worth noting that unmodified OCNT shows moderate activity in producing H 2 O 2 with 55% FE that is inferior to both CoPc-OCNT and CuPc-OCNT, indicating that metal sites in TMPc-OCNT are mainly responsible to the selectivity of H 2 O 2 production. To demonstrate the effect of O coordination on the Co sites, O-containing groups on OCNT are removed by reductive thermal treatment to prepare CNT-H supported CoPc (CoPc-CNT-H). After the substantial elimination of O-containing groups from OCNT (confirmed by XPS in Supplementary Fig. 29 ), only 0.17% Co is loaded on the CNT-H support using the similar preparation method, which is lower than that on CoPc-OCNT (0.30%) and CoPc-oriCNT (0.48%, prepared using original CNT). Consequently, the CoPc-CNT-H exhibits poor H 2 O 2 electrosynthesis performance (65% FE at 100–170 mA cm − 2 ) than CoPc-OCNT and CoPc-oriCNT (96–98% and 67–83% FE at 100–200 mA cm − 2 ) (Supplementary Fig. 30 ). Although a higher Co loading, CoPc-oriCNT deliveries more inferior Faradaic efficiency for producing H 2 O 2 especially at larger currents compared to the CoPc-OCNT. It is inferred that there are moderately agglomerated CoPc molecules in the CoPc-oriCNT due to less strong interaction between Co sites and insufficient O-containing groups on oriCNT (Supplementary Fig. 29c ), which demonstrates the crucial contribution of sufficient O modification to catalytic Co centers to the two-electron ORR selectivity. Fig. 5: H 2 O 2 electrosynthesis performance in a flow-cell electrolyzer based on the gas-diffusion cathode. a, b Concentrations of H 2 O 2 directly outputted from electrolyzer and the Faradaic efficiency of FePc-OCNT, CoPc-OCNT, CuPc-OCNT, OCNT, CoPc-oriCNT or CoPc-CNT-H cathodes at 100 mA cm − 2 (Data points and error bars represent the average and standard deviation of data from triplicate parallel tests). c H 2 O 2 concentration, Faradaic efficiency and TOF values of CoPc-OCNT at 100, 120, 200 and 300 mA cm − 2 . d H 2 O 2 production rate of CoPc-OCNT compared with most advanced catalysts newly reported (data sources are provided in Supplementary Table 8 ). e Stability evaluation of CoPc-OCNT cathode for continuous electrosynthesis of H 2 O 2 at 200 mA cm − 2 in a chronopotentiometry test. (Cathodic working area of 1 cm − 2 , the catholyte of 1.0 M KOH (pH 13.7) is one-pass flowed out at a rate of 5 mL h − 1 to bring out the generated H 2 O 2 , while the anolyte of 0.5 M H 2 SO 4 was circled at a rate of 33 mL h − 1 ). Full size image Figure 5c shows that when increasing the current on the CoPc-OCNT cathode, the concentration of directly outflowed H 2 O 2 almost linearly increases from 366 to 1084 mM (3.7 wt%) that can meet the concentration requirement for disinfection or wastewater treatment applications [42] (3 wt% is generally sufficient). The CoPc-OCNT cathode can delivery ORR current density up to 300 mA cm − 2 with remarkable FE of 96–100% that is higher than that achieved by majority of electrocatalysts currently reported and is comparable to the best values reported by Wang et al. [36] , [43] (Supplementary Table 7 and Supplementary Fig. 31 ). To better understand the intrinsic activity, the turnover frequency (TOF) per metal site for H 2 O 2 production is calculated. The CoPc-OCNT catalyst presents current-dependent TOF values that reach up to 649–1921 min − 1 at 100–300 mA cm − 2 , demonstrating superior activity of the Co sites to Cu or Fe sites (Supplementary Figs. 32 , 33 ). Significantly, the heterogeneous H 2 O 2 electrosynthesis method shows great potential in maximizing the intrinsic activity of catalysts compared to homogeneous ORR that relies on Co-based molecular catalysts in organic system (limited TOF even at large overpotentials) [44] . The results from the current study show continuous H 2 O 2 production in high-concentration, while which remains a great challenge for homogeneous molecular catalysis process that also suffers from H 2 O 2 separation from the catalyst. Additionally, the CoPc-OCNT delivers a remarkable H 2 O 2 production rate of 3892–11,527 mmol h − 1 g cat − 1 under the current densities of 100–300 mA cm − 2 (Supplementary Fig. 34 ), higher than the values reported to the best of our knowledge (Fig. 5d and Supplementary Table 8 ). As shown in Fig. 5e , the continuous 30 h electrosynthesis of H 2 O 2 at 200 mA cm − 2 stably produces H 2 O 2 at a concentration of 677–755 mM at a remarkable FE of 91–100%, demonstrating the electrochemical stability of the CoPc-OCNT electrode. In contrast, the activity and stability of CuPc-OCNT declines rapidly with increasing current, which might be ascribed to less robust bonding of CuPc on OCNT (Supplementary Fig. 32 ). We investigate the H 2 O 2 electrosynthesis performance of CoPc-OCNT catalyst in less alkaline electrolyte (0.01 M KOH), which shows 97% H 2 O 2 FE at 10 mA cm − 2 , but the FE drops to 27% at 20 mA cm − 2 due to large overpotential (Supplementary Fig. 35a ). The cell voltage can be significantly reduced by increasing electrolyte concentration or shortening the electrode distance to reduce solution resistance (Supplementary Figs. 35 , 36 ). Results show that the cell voltage can be markedly reduced even in 0.01 M KOH, and the current density for H 2 O 2 production is obviously lifted (Supplementary Fig. 35 ). When using 1 M KOH+0.5 M H 2 SO 4 or 1 M KOH as catholyte and anolyte, the H 2 O 2 FE are 83% and 75% at 1100 mA, and the partial H 2 O 2 currents can reach 913 and 823 mA, respectively (Fig. 6a ). The electrosynthesis process consumes an electric energy of 0.20–0.34 kWh for producing per kg 3 wt% H 2 O 2 in the small reactor (Supplementary Fig. 37 , calculations are described in Method) that is reduced to 0.12–0.28 kWh by the upgrading of the electrolyzer configuration, showing high-efficiency electrical energy conversion into valuable chemicals. Furthermore, the feasibility studies of scalable catalytic material preparation are explored, based on the simplicity of the CoPc-OCNT catalyst synthesis compared to the catalysts typically prepared by high-temperature carbonization. Five types of highly conductive, commercially available carbon materials are adopted as the supports for CoPc after introducing O-containing groups via the similar oxidization treatment to that of OCNT (Supplementary Figs. 38 , 39 ). CoPc-OVX (Cabot VXC72) and CoPc-OAB (acetylene black) catalysts show higher FE of 85–98% for H 2 O 2 production at 100–170 mA cm − 2 compared to CoPc-OBP (black pearl 2000), CoPc-OECP (Ketjenblack ECP-600JD) and CoPc-OYP (Kurary YP-80F) (Supplementary Fig. 40 ). CoPc-OVX and CoPc-OAB can produce about 330 and 550 mM H 2 O 2 at 100 and 150 mA cm − 2 that are higher than that on CoPc-OBP, CoPc-OECP and CoPc-OYP. The performance of H 2 O 2 electrosynthesis is closely related to the Co loading, and the best activity is achieved at a moderate loading while insufficient or excessive Co loading would degrade the activity and selectivity due to limited catalytic sites or CoPc aggregation. It’s worth noting that 0.2‒0.6 at% CoPc loadings on OCNT or commercial carbon materials approach the theoretical upper limit value of 0.6 at% that is estimated based on the densest monodisperse packing of CoPc on OCNT (described in Supplementary Fig. 41 ), where the space of adjacent Co sites is far enough to prevent the CoPc from aggregating and thus favor the two-electron ORR over the four-electron process. The results not only prove the wide versatility of the design of metal single-site catalysts, but also demonstrate the feasibility for scalable catalyst manufacture that is not limited by specific starting carbon materials. Furthermore, it is promising to prepare the high-density O-modified Co-(pyrrolic N) 4 sites to improve the activity for H 2 O 2 production by using the CoPc and commercial carbon materials as raw materials in further studies [24] , [25] . Fig. 6: Acidic electrosynthesis H 2 O 2 performance and Fenton applications. a, b H 2 O 2 electrosynthesis employing 1 M KOH+0.5 M H 2 SO 4 , 1 M KOH+1 M KOH, 0.3 M K 2 SO 4 +0.3 M K 2 SO 4 (pH 7.2 or 1.5) as catholyte and anolyte in the bigger flow-cell electrolyzer (test conditions: cathodic working area of 4 cm − 2 , catholyte and anolyte flow rates of 82–100 mL h − 1 ). c Pollutant removal and TOC removal efficiency by the flow-cell Fenton system. (Test conditions: 500 mA current, effluent H 2 O 2 rate of 72 mL h − 1 synthetic wastewater: 10 mg  L − 1 phenol, bisphenol A or levofloxacin and 1 mM Fe 2+ , flow rate of 700 mL h − 1 real coking wastewater: initial TOC of 44.1 mg L − 1 , 5 mM Fe 2+ dosage, flow rate of 140 mL h − 1 . ). Full size image The electrosynthesis of H 2 O 2 is also explored in different pH for satisfying specific on-site applications related with environmental remediation that requires for acidic H 2 O 2 , such as Fenton reaction only effectively works pH ~3. When using 0.1 M K 2 SO 4 catholyte and 0.5 M H 2 SO 4 anolyte, about 70 mM acidic H 2 O 2 can be produced at 20 mA cm −2 with 92% FE (Supplementary Fig. 42 ). To avoid additional potential differences brought by different electrolytes, we use a neutral or acidic electrolyte as both catholyte and anolyte to evaluate the performance of H 2 O 2 electrosynthesis on CoPc-OCNT. In the bigger reactor, it can achieve 461–748 mA partial H 2 O 2 currents with 75–92% FE at pH 1.5 and 375–607 mA partial H 2 O 2 currents with 76–94% FE at pH 7.2 (Fig. 6a ), which satisfy the concentration requirement from homogeneous or heterogeneous Fenton technology for wastewater treatment [45] , [46] . Notably, the CoPc-OCNT electrode shows exceptional high partial H 2 O 2 currents in acidic electrolytes with the addition of 0.3 M K + , while majority of carbon-based catalysts show low FE for H 2 O 2 production at current density over 50 mA cm − 2 . The performance enhancement is likely related to the effects of metal cations and drastic increase in local pH on electrode interface. The addition of metal cations was demonstrated to prevent further reduction of generated H 2 O 2 to H 2 O by squeezing away the protons, thus promoting H 2 O 2 selectivity [47] . The drastic increase in local pH on electrode–electrolyte interfaces due to the depletion of H + , especially when applying a current density over 100 mA cm − 2 , should also contribute to the enhanced H 2 O 2 current density [48] . The experimentally observed pH increasements of effluent catholyte during electrosynthesis of H 2 O 2 also confirm an increase in the pH (Fig. 6b ). We highlight that such electrocatalytic reaction interfaces including metal cations and pH gradients are difficult to be accurately modelled by the DFT approach in this study based on purely thermodynamic analysis. Advanced computational methods, such as ab initio molecular dynamics simulations, are the potential tools to better describe and simulate the electrocatalytic properties of catalytic materials under real experimental conditions by considering the effects of solvent and ions and the kinetic information after a preliminary screening on the two-electron ORR catalysts [24] , [25] , [47] , [49] . We built a flow-cell system combining electrosynthesis of H 2 O 2 and the Fenton reaction for wastewater treatment, which shows almost 100% removal of the biodegradable pollutants with a treatment capacity of 700 mL h − 1 , wherein 40–52% total organic carbons (TOC) can be converted into CO 2 (Fig. 6c ). This flow-cell Fenton system also shows good performance for real coking wastewater treatment with almost 90% TOC removal. The 12 h acidic H 2 O 2 electrosynthesis at 500 mA for refractory organic pollutant degradation and wastewater treatment by cooperating with the Fenton reaction demonstrates the potential in actual small-scale applications. In summary, the ORR volcano plot with Δ G *OOH as a key descriptor is established by DFT calculations to screen for highly selective two-electron electrocatalyst among TMPc catalysts. The Δ G *OOH values of TMPc are associated with the d-band center of TM, which accounts for the Δ G *OOH on CoPc being much closer to the peak of the volcano. The O dopant at the defective carbon site is demonstrated to modify the local electronic structure of the Co center in CoPc and helps achieve the Δ G *OOH closest to the peak of the volcano. The prepared CoPc-OCNT catalyst with the O-modified Co-(pyrrolic N) 4 configuration delivers high activity and H 2 O 2 selectivity in both alkaline and neutral electrolytes, verifying the theoretically predicted activity-volcano trend for the two-electron ORR. The industrial-relevant current densities up to 300 mA cm − 2 with 96–100% FE are achieved for continuous H 2 O 2 production at a record rate of 11,527 mmol h − 1 g cat − 1 in a flow-cell electrolyzer. The high H 2 O 2 production capacity at industrial-relevant currents is meaningful to help reduce infrastructure cost for promising scalable applications of H 2 O 2 electrosynthesis. Furthermore, this study demonstrates the versatility of the metal single-site catalyst design using various commercial carbons as starting materials and high applicability for H 2 O 2 electrosynthesis, presenting a promising potential in future large-scale H 2 O 2 manufacture and in-situ wastewater treatment and disinfection. Computational details Density functional theory calculations were conducted using the Vienna Ab-initio Simulation Package (VASP 5.4.4 version) [50] . The electron-ion interactions and electron exchange-correlation interactions are described by the projector augmented wave (PAW) potential and Perdew-Burke-Ernzerhof (PBE) functional with the generalized gradient approximation (GGA) method [51] , [52] . The structural models of TMPc, OCNT and TMPc-OCNT were constructed in a cell with lattice parameters of 17 Å × 17 Å × 20 Å (Supplementary Figs. 1 , 2 and 5 ). The k -point meshes of (1 × 1 × 1) was set. The spin polarization effect was considered for all calculations expect for OCNT. The cutoff energy of plane wave was set at 420 eV. All structural configurations were optimized until the forces on each atom were converged to less than 1 × 10 − 2 eV Å − 1 . Total free energy changes between two steps were less than 1 × 10 − 5 eV atom − 1 in electronic relaxation. The two-electron ORR pathway is described as the following steps: 
    ∗+O_2(g)+H^++e^-→*OOH
 (1) 
    ∗OOH+H^++e^-→∗+H_2O_2
 (2) where * and *OOH denote an unoccupied active site and adsorbed *OOH intermediate, respectively. Gibbs free energy (Δ G ) for each step at the given potential U was calculated by the following equation: [14] , [53] 
    G= E+ ZPE+U_0→ T-T× S+eU
 (3) where Δ G represents the free energy that is equal to the calculated Δ E after being corrected by zero-point energies (Δ ZPE ) and entropic contributions (Δ U 0→T – T × ΔS ) of adsorbates at 298.15 K. Δ E is the electronic energy difference between reactants and products for each step. These correction items can be conveniently calculated using a VASPKIT code [54] . U is the electrode potential versus reversible hydrogen electrode (vs RHE). It is worth pointing out that G (H + ) is calculated by the equal of G (H + )=0.5 G (H 2 ) – G ( e ) (pH=0, U =0 V), and G (O 2 ) is calculated by the equal of 2 G (H 2 ) + G (O 2 ) – 2 G (H 2 O) = −4.92 eV. During the two-electron ORR process, the limiting step is determined by both *OOH formation (Eq. ( 1 )) and *OOH removal (Eq. ( 2 )) from the catalytic sites. The theoretical overpotential is demonstrated to be a function of the *OOH binding energy, thus the limiting potential can be expressed as: [11] 
    U_L1=- G_∗OOH+4.92
 (4) 
    U_L2=G_∗OOH-3.52
 (5) Chemicals and materials Commercial CNT powder (L-MWNT-2040) was purchased from Shenzhen Nanotech Port Co., Ltd. (Shenzhen, China). Cobalt phthalocyanine (CoPc, >95%), copper phthalocyanine (CuPc, >90.0%), phthalocyanine iron(II) (FePc, >98.0%), phthalocyanine (Pc, >93.0%), Ce(SO 4 ) 2 (99.9%), KOH (>95%) and K 2 SO 4 (99%) were bought from Aladdin Co., Ltd. (Shanghai, China). N,N-dimethylformamide (DMF) was purchased from Bodi Chemical Reagent Co., Ltd, China. Nafion solution (5 wt%) was purchased from Du Pont Co., Ltd. Isopropanol was purchased from Tianjin Fuyu Fine Chemicals Co., Ltd. (China). Teflon-treated carbon fiber paper (HCP120) served as the support of GDE was provided by Hesen Electrical Co., Ltd. (Shanghai, China). Catalyst preparation The OCNT material was prepared by chemically creating oxygen functional groups on the surface of original CNT, which was fulfilled by the oxidization treatment using concentrated nitric acid. In a typical operation, 3 g CNT power was homogeneously dispersed in 68 wt% HNO 3 (150 mL) under continuous magnetic stirring. The oxidization treatment was conducted at 140 °C for 12 h, followed by water washing and drying. It is important to note that the evaporation of concentrated HNO 3 and the decomposition products should be carefully treated via ice water condenser. In this process, the possible metal impurities (such as Fe, Ni, Cu, Co) on the surface of CNT would be removed after intensive acid etching. CoPc-OCNT, CuPc-OCNT, FePc-OCNT and Pc-OCNT catalysts were prepared using a simple impregnation method at room temperature. Typically, CoPc, CuPc, FePc or Pc (20 mg) molecules were dissolved in strong polar solvent of DMF (100 mL), followed by dropwise adding into the OCNT/DMF mixture (200/250 mg/mL) under rigorous stirring. The assembly process of phthalocyanines molecules and the OCNT support was conducted for 20 h, followed by separation and freeze-drying treatments. By adjusting the mass percent ratio of CoPc and OCNT using 10, 20, 30 or 40 mg CoPc with fixed 200 mg OCNT, CoPc-OCNT-5, CoPc-OCNT-10, CoPc-OCNT-15, and CoPc-OCNT-20 were prepared. As a comparison, CNT-H was prepared by removing the oxygen groups on OCNT under the reductive H 2 atmosphere at 800 °C for 2 h. A control sample of CoPc-CNT-H was synthesized using the CNT-H support at 10% mass percent ratio of CoPc and CNT-H. Similarly, CoPc-ori-CNT was prepared using the original CNT as support. Catalyst characterization The morphology of catalysts was observed by SEM (Hitachi S-4800) and TEM (Thermo-Tecnai G2 F30 S-Twin). The oxygen functional groups on OCNT and chemical constitutes of TMPc-OCNT were identified by FT-IR (RRUKER, VERTEX 70) and XPS (Thermos K-Alpha+ instrument with Al Kα X-ray excitation source). The phase structure was measured by XRD (Smartlab 9 kW, Nippon Neoku Electric Co. Ltd., Japan) and Raman (laser confocal microscopy Raman with laser excitation at 532 nm). The surface area and pore characteristics were assessed using N 2 adsorption-desorption measurements (Quantachrome, Autosorb-IQ-C). The metal loadings of TMPc-OCNT were detected by XPS and inductively coupled plasma-mass spectrometry (ICP-MS, PerkinElmer, Nex ION 300D). The XAS was collected on the beamline BL01C1 at National Synchrotron Radiation Research Center (NSRRC), and the radiation was monochromatized by a Si (111) double-crystal monochromator. Ceshigo Research Service (Chengdu, China) provided the technical support for the data analysis of XANES and EXAFS that were processed using the Athena software [55] . Electrochemical measurements The ORR performance of TMPc-OCNT catalysts was studied by RRDE device (AFMSRCE type, Pine, Physicochemical Co. Ltd. (Hong Kong)). Firstly, 2 mg of catalyst powder was well-dispersed in the mixture that consists of 0.9 mL H 2 O, 0.1 mL isopropanol and 20 μL of Nafion (5 wt%) via ultrasonication for 30 min for achieving the catalyst ink. The Pt counter electrode and Ag/AgCl reference electrode were used coupled with RRDE to construct the three-electrode system. The potential was normalized by converting to RHE according to the equation of E vs RHE= E vs Ag/AgCl+0.2+0.0591×pH. The potential versus RHE was adopted unless otherwise specified. The polarization current on the disk electrode and the H 2 O 2 oxidation current on Pt ring electrode (fixed potential at 1.35 V vs RHE) were collected in O 2 and Ar-saturated 0.01 M KOH electrolyte (pH 11.9) and 0.1 M K 2 SO 4 (pH 7.2). The scan rate was set at 10 mV s − 1 and the rotating speed was set at 1600 rpm. The collection efficiency N of H 2 O 2 of the Pt ring electrode was calibrated to be 39%, which is theoretically based on one-electron reversible redox conversion of ferrocyanide/ferricyanide species [56] , [57] . It should be mentioned that the actual ORR current ( I R ) and H 2 O 2 oxidation current ( I R ) were obtained by subtracting the values obtained in Ar-saturated solution from that in O 2 condition. Based on the corrected currents, the H 2 O 2 selectivity is calculated by the Eq. ( 7 ) of 
    _2_2(%)=200×I_//I_+I_/
 (6) Electrode preparation and H 2 O 2 electrosynthesis The electrodes were prepared by loading as-synthesized TMPc-OCNT catalysts on GDE. In a typical process, 10 mg of catalyst was dispersed in the mixture that consists of 0.8 mL H 2 O, 0.2 mL isopropanol and 50 μL of Nafion (5 wt%) to form catalyst ink. 50 μL of catalyst ink was coated on GDE by hand-painting, followed by drying treatment at 40 o C. The catalyst loading is about 0.5 mg cm − 2 . Pt foil was used as the counter electrode to construct a two-electrode system for electrochemical H 2 O 2 production. The proton exchange membrane (Nafion 117) was used to separate the cathode and anode. The H 2 O 2 electrosynthesis was carried out at the constant currents using two types of flow-cell electrolyzers shown in Supplementary Figs. 28 and 36 . When employing the small reactor with a working area of 1 cm − 2 , KOH electrolyte (0.01, 0.1, 0.2, 0.5 or 1.0 M) was used as the catholyte with one-pass flow rate of 5 mL h − 1 to bring out the generated H 2 O 2 , and the anolyte of 0.5 M H 2 SO 4 was cycled at a rate of 33 mL h − 1 . Pure O 2 was supplied to the cathode side faced to the gas chamber at a flow rate of 20 mL min − 1 that was controlled by a mass flow controller (Sevenstar D07, China). The constant currents were provided by a workstation (Chenhua CHI760E, Shanghai, China). When employing the bigger reactor with a working area of 4 cm − 2 , the catholyte was one-time outflowed at a rate of 80–100 mL h − 1 , while the anolyte was cycled at the same flow rate. The flow rate of pure O 2 was controlled at 30 mL min −1 . The couples of 0.01 M KOH+0.5 M H 2 SO 4 , 0.1 M KOH+0.5 M H 2 SO 4 , 1 M KOH+0.5 M H 2 SO 4 , 1 M KOH+1 M KOH, 0.3 M K 2 SO 4 +0.3 M K 2 SO 4 (pH 7.2 or 1.5 that is adjusted using H 2 SO 2 ) were used as catholyte and anolyte to estimate the performance of H 2 O 2 electrosynthesis. The constant currents were provided by a direct-current power supply. The H 2 O 2 concentration was measured by the cerium sulfate titration method based on the stoichiometry of 2 Ce 4+ + H 2 O 2 = 2 Ce 4+ + 2 H + + O 2 . In a typical operation, 10 μL of H 2 O 2 solution outflowed from the reactor was added into the certain amount of Ce 4+ solution to reduce Ce 4+ to Ce 3+ . The Ce 4+ concentration can be detected by spectrophotometry at 316 nm. Thus, we calculated H 2 O 2 concentration via the equation of: 
    C(_2_2)=[_0(^4+)-C(^4+)]× V(^4+)/2× V(_2_2)
 (7) It should be noted that the consumed volume ( \(V({{{\mbox{Ce}}}}^{4+})\) , mL) of Ce 4+ solution (the initial concentration \({{{\mbox{C}}}}_{0}({{{\mbox{Ce}}}}^{4+})\) is 1 mM) for detecting H 2 O 2 was at the range of 5–40 mL, which was far larger than \(\,V({{{\mbox{H}}}}_{2}{{{\mbox{O}}}}_{2})\) of the H 2 O 2 solution (10 μL). Otherwise, this simplified equation above needs to be corrected. Electricity consumption calculation The electricity consumption for per kg H 2 O 2 (3 wt%) production is calculated according to the equation of 
    E=30× U× I/C×(_2_2)× v
 (8) E represents electricity consumption (kWh kg − 1 3 wt% H 2 O 2 ), I and U represent applied current and cell potential (V, A), respectively, and C , M(H 2 O 2 ) and v represent H 2 O 2 concentration (mol L − 1 ), H 2 O 2 molecular weight (34 g mol − 1 ) and flow rate, respectively. Reporting summary Further information on research design is available in the Nature Portfolio Reporting Summary linked to this article.